ATP-triggered anticancer drug delivery Stimuli-triggered drug delivery systems have been increasingly used to promote physiological specificity and on-demand therapeutic efficacy of anticancer drugs. Here we utilize adenosine-5'-triphosphate (ATP) as a trigger for the controlled release of anticancer drugs. We demonstrate that polymeric nanocarriers functionalized with an ATP-binding aptamer-incorporated DNA motif can selectively release the intercalating doxorubicin via a conformational switch when in an ATP-rich environment. The half-maximal inhibitory concentration of ATP-responsive nanovehicles is 0.24 μM in MDA-MB-231 cells, a 3.6-fold increase in the cytotoxicity compared with that of non-ATP-responsive nanovehicles. Equipped with an outer shell crosslinked by hyaluronic acid, a specific tumour-targeting ligand, the ATP-responsive nanocarriers present an improvement in the chemotherapeutic inhibition of tumour growth using xenograft MDA-MB-231 tumour-bearing mice. This ATP-triggered drug release system provides a more sophisticated drug delivery system, which can differentiate ATP levels to facilitate the selective release of drugs. Nanocarrier-based drug delivery systems (DDSs) offer new opportunities to improve bioactivity and prolong bioavailability of drugs for cancer therapy [1] , [2] , [3] , [4] . To further enhance biological specificity and therapeutic efficacy, significant efforts have been devoted to explore active targeting [5] and stimuli-responsive DDSs [6] , which specifically accumulate at the tumour site and are stimulated to release drugs within tumour cells. These stimuli can be a variety of external signals, such as temperature [7] , light [8] , magnetic field [9] , ultrasound [10] and electric current [11] , as well as physiological factors, such as pH [12] , redox potential [13] , enzymatic activities [14] , [15] and glucose levels [16] , [17] . A number of nanosystems including liposomes [18] , polymeric nanoparticles [19] and inorganic particles [20] have been developed to apply these triggering cues to tailor pharmacokinetics and enhance delivery efficiency. For example, acid-sensitive species have been widely incorporated in intracellular delivery vehicles that undergo an endocytosis pathway, thereby allowing drugs to be readily released in acidic compartments [12] . The gradient of reduced glutathione enables polymeric nanogels crosslinked with glutathione-cleavable disulphides to efficiently release payloads inside cells [21] . The proteases highly expressed in specific tumour microenvironments facilitate nanocarriers consisting of relevant peptidyl substrates to release drugs on demand [14] . In this study, we report that ATP, the most abundant ribonucleotide used in cells as a coenzyme, can serve as a new trigger for the controlled release of anticancer drugs both in vitro and in vivo . As the ‘molecular unit of currency’ of intracellular energy transfer, ATP transports chemical energy within cells to support metabolism [22] . ATP is present in low concentrations (<0.4 mM) in the extracellular environment, but is relatively concentrated within the intracellular cytosol (1–10 mM) [23] , [24] , [25] , [26] . Within cells, ATP provides energy to the cellular metabolism by breaking a phosphoanhydride bond. The prominent difference in the ATP level between the extracellular and intracellular environments is the biological rationale for design of ATP-mediated drug release systems, which remain elusive [27] . Recently, Biswas et al . [28] applied the hydrolysis of intracellular ATP into ADP to trigger conformational variation of the chaperonin units in the supramolecular nanotubes, which subsequently caused the disassembly of the tubes and release of the guests. Using a different strategy, we envision that ATP-responsive nanosystems can be functionalized with ATP-binding aptamers, which are specifically recognized and activated by ATP and directly promote the release of preloaded anticancer drugs. The nanocarriers can selectively release the drug via a conformational switch under an ATP-rich environment for enhanced cytotoxicity and apoptosis. On a combination of passive and active targeting effects, the system presents an improvement in the chemotherapeutic inhibition of tumour growth in mice. We designed a nanocarrier comprised of DNA, protein and polysaccharide. As shown in Fig. 1a , the final formulation (designated nanogel) is mainly comprised of three distinct functional constituents: an ATP-responsive DNA motif with doxorubicin (Dox), protamine and a hyaluronic acid (HA)-crosslinked shell. The DNA scaffold consists of the ATP aptamer and its complementary single-stranded DNA (cDNA), the structure of which has been previously used to detect ATP [29] , [30] , [31] , [32] . The GC pairs of the DNA motif provide faithful loading sites for Dox, a model chemotherapeutic drug used to treat a wide spectrum of cancers, including breast cancer, ovarian cancer and acute leukaemia. In the presence of ATP, the tertiary structure of the ATP aptamer is stabilized, which causes the DNA duplex to dissociate and thereby liberates cDNA. In our strategy, this structural change from the duplex to the tertiary aptamer structure (duplex-to-aptamer) results in the intercalated Dox to be released from the duplex ( Fig. 1b ). Protamine is positively charged and is applied to compress the negatively charged DNA scaffold into a cationic core complex, which has enhanced cell penetration, endosomal escape and nuclear targeting effects [33] . Anionic HA is coated on the core complex to form a protective shell, and also supports active tumour-targeting ligands to bind the receptors, such as CD44 and RHAMM, which are overexpressed on the cell surface of several tumours [34] . In addition, hyaluronidase (HAase) [35] , rich in various malignant tumour matrices and the tumour cellular endocytic vesicles including endosomes and lysosomes (endolysosomes) [36] , leads to the degradation of the HA shell and allows the exposure of the cationic complex to facilitate intracellular delivery. To obtain the compact ‘gel’ structure [37] , protamine and HA are modified with acrylamide (designated m -protamine) and acrylate groups (designated m -HA), respectively. The final nanogels are constructed by photocrosslinking via UV irradiation. 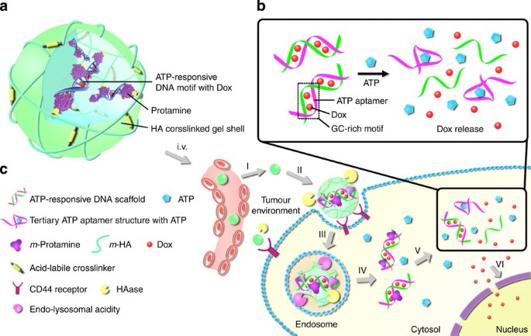Figure 1: Schematic design of the ATP-triggered Dox release system. (a) The main components of Dox/NG: ATP-responsive DNA motif with Dox, protamine and a HA-crosslinked gel shell. (b) Mechanism of ATP-triggered release of Dox based on the structural change of duplex-to-aptamer. (c) ATP-responsive delivery of Dox by Dox/NG to nuclei for the targeted cancer therapy. I, accumulation of Dox/NG at the tumour site through passive and active targeting; II, specific binding to the overexpressing receptors on the tumour cells and degradation of HA shell by HAase rich in the tumour extracellular matrix; III, receptor-mediated endocytosis; IV, endosomal/lysosomal escape; V, ATP-triggered Dox release in the cyotosol; VI, accumulation of Dox in the nucleus. Figure 1: Schematic design of the ATP-triggered Dox release system. ( a ) The main components of Dox/NG: ATP-responsive DNA motif with Dox, protamine and a HA-crosslinked gel shell. ( b ) Mechanism of ATP-triggered release of Dox based on the structural change of duplex-to-aptamer. ( c ) ATP-responsive delivery of Dox by Dox/NG to nuclei for the targeted cancer therapy. I, accumulation of Dox/NG at the tumour site through passive and active targeting; II, specific binding to the overexpressing receptors on the tumour cells and degradation of HA shell by HAase rich in the tumour extracellular matrix; III, receptor-mediated endocytosis; IV, endosomal/lysosomal escape; V, ATP-triggered Dox release in the cyotosol; VI, accumulation of Dox in the nucleus. Full size image After intravenous injection, the nanogel is expected to accumulate at tumour sites as a result of passive and active targeting effects. HAase degrades the HA shell, thereby exposing the complex of protamine with the Dox-intercalated duplex (Dox/Duplex). The protamine component promotes endosomal escape of the complex, allowing the efficient transport of Dox/Duplex into the cytosol. Dox/Duplex dissociates at a significantly higher ATP level in the cytosol compared with the extracellular fluid, thereby yielding the release of intercalating Dox, which eventually accumulates in the nuclei to produce cytotoxicity and apoptosis ( Fig. 1c ). This ATP-triggered drug release system offers new avenues for exploration of more sophisticated DDSs, which integrates with tumour metabolism for controlled release of anticancer drugs. ATP-triggered Dox release from duplex We first designed a DNA scaffold by hybridizing an ATP aptamer and its cDNA ( Supplementary Table 1 , Supplementary Methods ), which has a 27-base pair with GC-rich motif for anthracycline-contained Dox loading [38] . To evaluate the amount of Dox molecules loaded into the ATP-Duplex, we measured Dox intercalation by monitoring Dox fluorescence intensity changes. When a fixed concentration of Dox was incubated with an increasing molar ratio of the DNA duplex, a sequential decrease was found in the fluorescence intensity of Dox ( Fig. 2a ) due to the initiation of förster resonance energy transfer between Dox molecules when intercalated into the DNA duplex [39] , [40] . A maximum quenching efficacy was achieved when the molar ratio of duplex to Dox was 0.5. To investigate the ATP-responsive characteristics of the duplex, Dox/Duplex was incubated at 0.4 mM and 4 mM ATP concentrations, which represent the typical ATP level in the extracellular fluid and intracellular cytosol, respectively [23] , [24] , [25] , [26] . The dissociation of Dox/Duplex leads to the release of Dox, which can be estimated by detecting the recovery of the Dox fluorescence. As shown in Fig. 2b , a remarkable fluorescence recovery was observed in the presence of 4 mM ATP concentration compared with the 0.4 mM sample, indicating that Dox/Duplex is responsive to high concentrations of ATP. The fluorescence recovery ratio (( F NTP - F )/( F 0 − F )) showed that the Dox release from Dox/Duplex was ATP-concentration dependent ( Fig. 2c ), where F 0 is the fluorescence intensity of Dox in the Dox solution without the duplex, and F NTP and F are the fluorescence intensities of Dox in Dox/Duplex at the same Dox concentration as in the Dox solution in the presence and absence of ATP, respectively. The fluorescence recovery ratio was determined as 20 and 31% at ATP concentrations of 2 and 4 mM, about fourfold and sevenfold greater than that at an ATP concentration of 0.4 mM, respectively. In contrast, negligible changes were found in the fluorescence recovery ratio of Dox/Duplex after incubation with the analogues of ATP such as cytidine triphosphate, guanosine triphosphate and uridine triphosphate, suggesting that the ATP aptamer-functionalized Dox/Duplex had a good selectivity to ATP compared with its analogues, which were unable to release Dox even at high levels. Furthermore, we took Dox-loaded control duplex (Dox/cDuplex) [31] that had the same length but was not responsive to ATP as a reference ( Supplementary Table 1 and Supplementary Fig. 1 ). The fluorescence recovery ratio of Dox/Duplex was about fivefold of that of Dox/cDuplex in the presence of a 4 mM ATP concentration ( Fig. 2d ), substantiating that the ATP aptamer endowed Dox/Duplex with the ATP-responsive drug release capability. Taken together, Dox/Duplex, the ATP-responsive DNA motif encapsulating Dox, can be used to effectively release Dox via a duplex-to-aptamer structural change under elevated ATP concentrations, which provides a foundation for the construction of an ATP-responsive DDS. 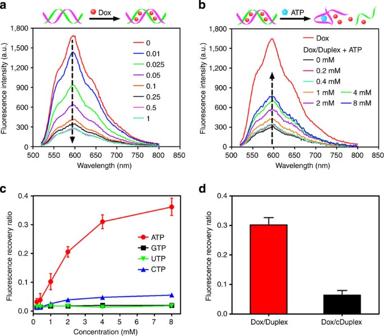Figure 2: ATP-triggered Dox release from duplex. (a) The fluorescence spectra of the Dox solution (1.33 μM) with increasing molar ratios of hybridized DNA duplex of ATP aptamer and its complementary single-stranded DNA (from top to bottom: 0, 0.01, 0.025, 0.05, 0.1, 0.25, 0.5, 1 equiv.) after 15 min of incubation in the HEPES buffer (5 mM). (b) The fluorescence spectra of Dox/Duplex (1.33 μM) at the molar ratio of duplex to Dox as 0.5 in the presence of different concentrations of ATP (0.2, 0.4, 1, 2, 4, 8 mM) after 15 min of incubation. (c) Fluorescence recovery ratios of Dox/Duplex in the presence of different concentrations of ATP, GTP, CTP and UTP (0.2, 0.4, 1, 2, 4, 8 mM). Error bars indicate s.d. (n=3). (d) Fluorescence recovery ratios of Dox/Duplex and Dox/cDuplex in the presence of 4 mM ATP. Error bars indicate s.d. (n=3). The fluorescence recovery ratio is indicated as (FNTP−F)/(F0−F), whereF0is the fluorescence intensity of Dox in the Dox solution without the duplex, andFNTPandFare the fluorescence intensities of Dox in Dox/Duplex at the same Dox concentration with the Dox solution in the presence and absence of NTP, including ATP, CTP, GTP and UTP, respectively. In (b–d), the buffer and salt condition is the HEPES buffer (5 mM) containing 10 mM MgCl2and 137 mM NaCl. CTP, cytidine triphosphate; GTP, guanosine triphosphate; UTP, uridine triphosphate. Figure 2: ATP-triggered Dox release from duplex. ( a ) The fluorescence spectra of the Dox solution (1.33 μM) with increasing molar ratios of hybridized DNA duplex of ATP aptamer and its complementary single-stranded DNA (from top to bottom: 0, 0.01, 0.025, 0.05, 0.1, 0.25, 0.5, 1 equiv.) after 15 min of incubation in the HEPES buffer (5 mM). ( b ) The fluorescence spectra of Dox/Duplex (1.33 μM) at the molar ratio of duplex to Dox as 0.5 in the presence of different concentrations of ATP (0.2, 0.4, 1, 2, 4, 8 mM) after 15 min of incubation. ( c ) Fluorescence recovery ratios of Dox/Duplex in the presence of different concentrations of ATP, GTP, CTP and UTP (0.2, 0.4, 1, 2, 4, 8 mM). Error bars indicate s.d. ( n =3). ( d ) Fluorescence recovery ratios of Dox/Duplex and Dox/cDuplex in the presence of 4 mM ATP. Error bars indicate s.d. ( n =3). The fluorescence recovery ratio is indicated as ( F NTP − F )/( F 0 − F ), where F 0 is the fluorescence intensity of Dox in the Dox solution without the duplex, and F NTP and F are the fluorescence intensities of Dox in Dox/Duplex at the same Dox concentration with the Dox solution in the presence and absence of NTP, including ATP, CTP, GTP and UTP, respectively. In ( b – d ), the buffer and salt condition is the HEPES buffer (5 mM) containing 10 mM MgCl 2 and 137 mM NaCl. CTP, cytidine triphosphate; GTP, guanosine triphosphate; UTP, uridine triphosphate. Full size image Preparation and characterization of ATP-responsive nanogels Dox/Duplex was mixed with m -protamine at an optimal mass ratio of 14:17 to prepare a positively charged Dox-loaded complex [41] (Dox/Complex) ( Fig. 3a and Supplementary Fig. 2 ). The complex was then added to the m -HA solution at a mass ratio of m -HA to m -protamine as 1:1 to obtain an HA-coated Dox/Complex (Dox/HA-Complex) with a negative charge ( Fig. 3b and Supplementary Figs 3 and 4 ). Ultimately, Dox-loaded nanogel (Dox/NG) was obtained by photocrosslinking Dox/HA-Complex with an acid-labile crosslinker glycerol dimethacrylate (GDA). Insignificant influence on the ATP response of Dox/Duplex was found after a short period of UV exposure ( Supplementary Fig. 5 ). The fluorescence of Dox was still quenched in the obtained Dox/NG ( Supplementary Fig. 6 ). As shown in Fig. 3c , the changes in the particle size and zeta potential from Dox/Duplex to Dox/NG suggested an efficient HA coating of the complex and the synthesis of Dox/NG, which had a resulting particle diameter of about 160 nm with a polydispersity index of 0.144 ( Supplementary Fig. 7 ) and a zeta potential of –20 mV. Transmission electron microscope (TEM) imaging further confirmed a spheroid structure of Dox/NG with a uniform particle size of about 150 nm ( Fig. 3d ). 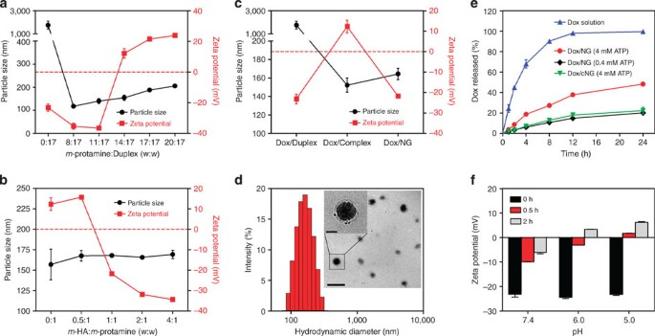Figure 3: Characterization of ATP-responsive nanogels. (a) The particle size and zeta potential of Dox/Complex at different mass ratios ofm-protamine and duplex. Error bars indicate s.d. (n=3). (b) The particle size and zeta potential of Dox/HA-Complex at different mass ratios ofm-HA andm-protamine. Error bars indicate s.d. (n=3). (c) The particle size and zeta potential of Dox/Duplex, Dox/Complex and Dox/NG. Error bars indicate s.d. (n=3). (d) The hydrodynamic size of Dox/NG measured by dynamic light scattering. Inset: TEM image of Dox/NG (accelerating voltage: 80 kV). Scale bars are 100 nm (upper) and 500 nm (lower). (e)In vitrorelease of Dox/NG and Dox/cNG at different concentrations of ATP. Error bars indicate s.d. (n=3). (f) Changes in the zeta potential of Dox/NG incubated with 0.5 mg ml−1HAase at different pH values for different time. Error bars indicate s.d. (n=3). Figure 3: Characterization of ATP-responsive nanogels. ( a ) The particle size and zeta potential of Dox/Complex at different mass ratios of m -protamine and duplex. Error bars indicate s.d. ( n =3). ( b ) The particle size and zeta potential of Dox/HA-Complex at different mass ratios of m -HA and m -protamine. Error bars indicate s.d. ( n =3). ( c ) The particle size and zeta potential of Dox/Duplex, Dox/Complex and Dox/NG. Error bars indicate s.d. ( n =3). ( d ) The hydrodynamic size of Dox/NG measured by dynamic light scattering. Inset: TEM image of Dox/NG (accelerating voltage: 80 kV). Scale bars are 100 nm (upper) and 500 nm (lower). ( e ) In vitro release of Dox/NG and Dox/cNG at different concentrations of ATP. Error bars indicate s.d. ( n =3). ( f ) Changes in the zeta potential of Dox/NG incubated with 0.5 mg ml −1 HAase at different pH values for different time. Error bars indicate s.d. ( n =3). Full size image To evaluate ATP-triggered Dox release characteristics, we investigated in vitro release profiles of Dox from Dox/NG in the presence and absence of ATP at 37 °C. Both Dox/NG and non-ATP-responsive Dox-loaded control nanogel (Dox/cNG), which consisted of the same components with Dox/NG except Dox/cDuplex, presented a sustained Dox release compared with the Dox solution ( Fig. 3e ). More importantly, in the presence of 0.4 mM ATP, only 6% of Dox was released from Dox/NG in the first 4 h and ~20% was released within 24 h. In the same buffer solution with 4 mM ATP, a level comparable to intracellular ATP levels, the release of Dox was dramatically accelerated. About 20% of Dox was released from Dox/NG in the first 4 h and more than 40% was released within 24 h. It is also noteworthy that the release of Dox from Dox/cNG (without ATP sensitivity) was slow even in the presence of 4 mM ATP. It is therefore implied that the ATP aptamer is essential for Dox/NG to recognize ATP concentration and allow the fast release of the intercalated Dox molecules in ATP-rich environments, and Dox remains entrapped in the inner cores of Dox/NG at low ATP concentrations. To demonstrate HA degradation by HAase [35] , the variation in the zeta potential of Dox/NG was monitored after incubation with HAase at different pH values over time. As shown in Fig. 3f , the zeta potential of Dox/NG sharply changed from highly negative (–23 mV) to less negative (–6 mV) after exposure to HAase for 2 h at pH 7.4. Moreover, the HA shell of Dox/NG crosslinked by GDA showed a pH-dependent degradation. Higher acidities had a concomitant enhancement on the degradation of the shell of Dox/NG. At 2 h, the zeta potential of Dox/NG continuously rose to +3 mV at pH 6.0 and +6 mV at pH 5.0, while Dox/NG still presented slightly negative charge of –6 mV at pH 7.4. Accordingly, the crosslinked HA shell of Dox/NG will be preferentially dissociated in the HAase-rich acidic tumour microenvironment and intracellular endolysosome to ‘turn off’ the protective function of HA and ‘turn on’ the penetrating activity of the protamine-based complex for efficient intracellular delivery. Intracellular ATP-triggered Dox release of Dox/NG We next investigated whether intracellular ATP could accelerate the release of Dox determined by the fluorescence recovery of Dox in the cells. To assess this, the human breast adenocarcinoma (MDA-MB-231) cells were incubated with Dox/cNG and Dox/NG for 2 h and the excess nanogels were thoroughly removed. The cells were then incubated with fresh culture medium for an additional 2 or 4 h. The amount of released Dox was evaluated by recording the fluorescence intensity of the whole cells. Dox fluorescence was observed during the first 2 h of the cellular uptake of Dox/NG at 37 °C ( Fig. 4a ), which resulted from the unquenched background fluorescence of Dox and the Dox released from Dox/NG [40] . Notably, Dox/NG presented a concomitant increase of fluorescence intensity with increasing incubation time of the cells. The fluorescence intensity had 30 and 49% significant increase after an additional 2 h and 4 h of incubation, respectively. However, the cells incubated with Dox/cNG showed no evident increase in the Dox fluorescence intensity. This prominent difference in the fluorescence intensity between cells incubated with Dox/NG and Dox/cNG suggested that Dox/NG was able to selectively liberate Dox in a more efficient manner based on the intracellular ATP level by ATP-responsive structural changes, relative to Dox/cNG that released Dox by passive diffusion. To further demonstrate the intracellular ATP concentration-dependent Dox release from Dox/NG, we inhibited the ATP production of the cells by physically lowering the temperature (4 °C) and adding a chemical inhibitor, iodoacetic acid (IAA) [42] , and subsequently monitored the fluorescence intensity after the treated cells were incubated with Dox/NG. Cell incubation at 4 °C and with IAA at 37 °C both led to a significant decrease in ATP generation within the cells ( Fig. 4b ). As expected, no remarkable release of Dox from Dox/NG was found in the cells that were incubated at 4 °C, nor with IAA at 37 °C for additional 2 h or 4 h ( Fig. 4c ), further confirming the intracellular ATP-mediated drug release capability of Dox/NG. 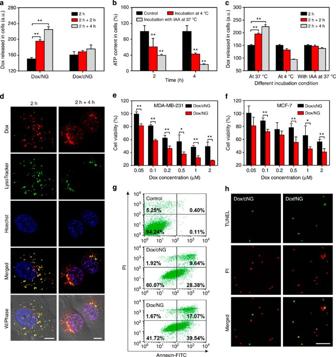Figure 4: Intracellular ATP-triggered Dox release. (a) Dox released in MDA-MB-231 cells of Dox/NG and Dox/cNG obtained using the flow cytometry. The cells were incubated with Dox/NG or Dox/cNG at 37 °C for 2 h, and subsequently incubated with fresh culture medium at 37 °C for additional 2 h or 4 h after removal of the excess nanogels. Error bars indicate s.d. (n=3). **P<0.01 (two-tailed Student’st-test). (b) The ATP content in MDA-MB-231 cells after different treatments. Error bars indicate s.d. (n=3). **P<0.01 compared with the control group (two-tailed Student’st-test). (c) Dox released in MDA-MB-231 cells of Dox/NG obtained using the flow cytometry. The cells were incubated with Dox/NG at 37 °C for 2 h, and then incubated with the fresh culture medium at 4 °C or with IAA at 37 °C for additional 2 h or 4 h after removal of the excess nanogels. Error bars indicate s.d. (n=3). **P<0.01 (two-tailed Student’st-test). (d) Intracellular delivery of Dox/NG on MDA-MB-231 cells at different time observed by CLSM. The cells were incubated with Dox/NG at 37 °C for 2 h, and further incubated with fresh culture medium at 37 °C for additional 4 h after removal of the excess nanogels. The late endosomes and lysosomes were stained by LysoTracker Green, and the nuclei were stained by Hoechst 33342. Scale bar is 10 μm. (e,f)In vitrocytotoxicity of Dox/cNG and Dox/NG on MDA-MB-231 (e) and MCF-7 cells (f) for 24 h. Error bars indicate s.d. (n=4). *P<0.05, **P<0.01 (two-tailed Student’st-test). (g) Flow cytometric analysis of MDA-MB-231 cell apoptosis induced by Dox/cNG and Dox/NG for 12 h using the Annexin V-FITC/PI staining. In each panel, the lower-left (Annexin V-FITC−, PI−), lower-right (Annexin V-FITC+, PI−) and upper-right (Annexin V-FITC+, PI+) quadrants represent the populations of live cells, early apoptotic cells and late apoptotic cells, respectively. The average population (%) in each quadrant is indicated by the numbers at the corner of the panels. (h) MDA-MB-231 cell apoptosis induced by Dox/cNG and Dox/NG for 20 h using the APO-BrdU TUNEL assay. Alexa Fluor 488-stained nick end label showed green fluorescence, and PI-stained nuclei showed red fluorescence. Scale bar is 100 μm. Figure 4: Intracellular ATP-triggered Dox release. ( a ) Dox released in MDA-MB-231 cells of Dox/NG and Dox/cNG obtained using the flow cytometry. The cells were incubated with Dox/NG or Dox/cNG at 37 °C for 2 h, and subsequently incubated with fresh culture medium at 37 °C for additional 2 h or 4 h after removal of the excess nanogels. Error bars indicate s.d. ( n =3). ** P <0.01 (two-tailed Student’s t -test). ( b ) The ATP content in MDA-MB-231 cells after different treatments. Error bars indicate s.d. ( n =3). ** P <0.01 compared with the control group (two-tailed Student’s t -test). ( c ) Dox released in MDA-MB-231 cells of Dox/NG obtained using the flow cytometry. The cells were incubated with Dox/NG at 37 °C for 2 h, and then incubated with the fresh culture medium at 4 °C or with IAA at 37 °C for additional 2 h or 4 h after removal of the excess nanogels. Error bars indicate s.d. ( n =3). ** P <0.01 (two-tailed Student’s t -test). ( d ) Intracellular delivery of Dox/NG on MDA-MB-231 cells at different time observed by CLSM. The cells were incubated with Dox/NG at 37 °C for 2 h, and further incubated with fresh culture medium at 37 °C for additional 4 h after removal of the excess nanogels. The late endosomes and lysosomes were stained by LysoTracker Green, and the nuclei were stained by Hoechst 33342. Scale bar is 10 μm. ( e , f ) In vitro cytotoxicity of Dox/cNG and Dox/NG on MDA-MB-231 ( e ) and MCF-7 cells ( f ) for 24 h. Error bars indicate s.d. ( n =4). * P <0.05, ** P <0.01 (two-tailed Student’s t -test). ( g ) Flow cytometric analysis of MDA-MB-231 cell apoptosis induced by Dox/cNG and Dox/NG for 12 h using the Annexin V-FITC/PI staining. In each panel, the lower-left (Annexin V-FITC − , PI − ), lower-right (Annexin V-FITC + , PI − ) and upper-right (Annexin V-FITC + , PI + ) quadrants represent the populations of live cells, early apoptotic cells and late apoptotic cells, respectively. The average population (%) in each quadrant is indicated by the numbers at the corner of the panels. ( h ) MDA-MB-231 cell apoptosis induced by Dox/cNG and Dox/NG for 20 h using the APO-BrdU TUNEL assay. Alexa Fluor 488-stained nick end label showed green fluorescence, and PI-stained nuclei showed red fluorescence. Scale bar is 100 μm. Full size image The intracellular delivery of Dox/NG in MDA-MB-231 cells was also explored using confocal laser scanning microscopy (CLSM). Dox/NG was demonstrated to bind to the CD44 receptor on the cell membrane ( Supplementary Fig. 8 ), followed by internalization via the clathrin-mediated pathway ( Supplementary Fig. 9 ) and subsequent transportation into the endosomes and lysosomes [43] , [44] . As shown in Fig. 4d , most of the endocytosed Dox/NG was located in the endolysosomes judged by the yellow fluorescence during the first 2 h of incubation. However, after an additional 4 h of incubation, the conspicuous dissociation of the broader red fluorescence and less green fluorescence suggested the endolysosomal escape of Dox/NG with the help of protamine, and led to a significant release of Dox resulting from the high cytosolic ATP level. Furthermore, the released Dox specifically accumulated into the nuclei, as evidenced by the magenta fluorescence characteristic of a cascade in apoptosis. The in vitro cytotoxicity of Dox/NG against two kinds of human breast adenocarcinoma cells, specifically MDA-MB-231 and MCF-7 cells, was evaluated by using the 3-(4,5-dimethylthiazol-2-yl)-2,5-diphenyltetrazolium bromide (MTT) assay. Dox/NG presented the significantly enhanced cytotoxicity compared with Dox/cNG towards both MDA-MB-231 and MCF-7 cells at all the Dox concentrations studied ( Fig. 4e,f ). IC 50 of Dox/NG was 0.24 μM on MDA-MB-231 cells and 0.80 μM on MCF-7 cells, which was remarkably lower than that of Dox/cNG, 1.1 μM on MDA-MB-231 cells and 2.9 μM on MCF-7 cells, respectively. Dox/NG also showed greater cytotoxicity than the Dox solution (IC 50 =0.30 μM) on MDA-MB-231 cells ( Supplementary Fig. 10 ) and Dox-loaded PEGylated liposomes (Dox/PEG-L) on both cancer cells ( Supplementary Fig. 11 ). Blank nanogels without Dox did not show toxicity within the tested range of concentrations ( Supplementary Fig. 12 ). It was suggested that the efficient intracellular release of Dox from Dox/NG compared with Dox/cNG provides higher cytotoxic activity towards the cancer cells. Furthermore, to demonstrate that Dox effectively released from Dox/NG could also induce elevated apoptosis, the Annexin V-FITC/PI apoptosis detection and the terminal deoxynucleotidyl transferase dUTP nick end labelling (TUNEL) assay were performed to compare the apoptosis-inducing capabilities of Dox/NG and Dox/cNG. Annexin V-FITC labels the phosphatidylserine sites that translocates to the extracellular membrane upon initiation of apoptosis, while PI labels the intracellular DNA in the late apoptotic cells where the plasma membrane has been compromised [45] , [46] . This combination allows the differentiation among the early apoptotic cells, the late apoptotic cells and the viable cells, which can be quantitatively determined by the flow cytometry [47] . The total apoptotic ratio of Dox/NG was 56.61% obtained by summation of the early apoptotic ratio of 39.54% and the late apoptotic ratio of 17.07%, which was much higher than 38.02% of Dox/cNG ( Fig. 4g ). In addition, during apoptosis, caspase 3 cleaves the inhibitor of caspase-activated deoxyribonuclease and produces nucleosomal DNA fragmentation [48] , which can be visualized with the TUNEL assay using CLSM [49] . MDA-MB-231 cells treated with Dox/NG showed more extensive apoptotic DNA fragmentation stained by the Alexa Fluor 488 as green fluorescence in comparison with that treated with Dox/cNG ( Fig. 4h ). These results confirmed that ATP-responsive Dox/NG is an effective intracellular nanocarrier delivery system for enhanced apoptosis-inducing activity. Tumour targeting and antitumour efficacy of Dox/NG To evaluate the tumour targeting capability of Dox/NG, the in vivo biodistribution of Cy5.5-labelled Dox/NG (Dox/Cy5.5-NG) administrated intravenously into the MDA-MD-231 tumour-bearing mice was investigated by a non-invasive near-infrared optical imaging technique. Dox/Cy5.5-NG presented a stronger fluorescence signal in the tumour region over a short time compared with Cy5.5-labelled Dox/Complex (Dox/Cy5.5-Complex) without the HA shell ( Fig. 5a ). As time increased, elevated fluorescence signals of Dox/Cy5.5-NG were found at the tumour site as compared with the normal tissues within 24 h post injection, indicating a notable tumour targeting effect of the nanogels. To further confirm the role of the interaction between CD44 receptors and HA in this high tumour targetability of the nanogels, a high dose of free HA was intravenously pre-injected prior to administration of Dox/Cy5.5-NG to block CD44-mediated binding of the nanogels on tumour tissue. As expected, the fluorescence signal of Dox/Cy5.5-NG significantly reduced at the tumour site after pre-injection of free HA into the mice ( Fig. 5a ). After 24 h post injection, the mice were immediately euthanized, and the tumours as well as normal tissues were harvested for ex vivo imaging. The fluorescence signal of Dox/Cy5.5-NG at the tumour site was significantly higher than that of Dox/Cy5.5-Complex and Dox/Cy5.5-NG pretreated with free HA ( Fig. 5b ), which was sextupled and tripled using quantitative region-of-interest analysis, respectively ( Fig. 5c ). In addition, the fluorescence signal at the tumour site was approximately double than that in the liver or kidney after injection of Dox/Cy5.5-NG for 24 h ( Fig. 5b,c ). 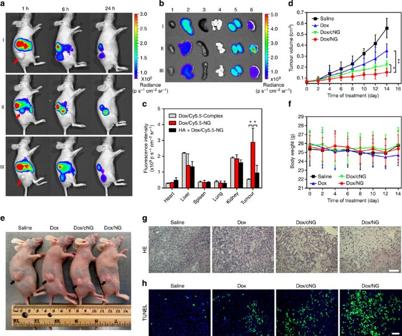Figure 5: Tumour targetability and antitumour activity. (a)In vivofluorescence imaging of the MDA-MB-231 tumour-bearing nude mice at 1, 6 and 24 h after intravenous injection of Dox/Cy5.5-Complex (I), Dox/Cy5.5-NG (II) and Dox/Cy5.5-NG with pre-injection of free HA (III) at Cy5.5 dose of 30 nmol kg−1. Arrows indicate the sites of tumours. (b)Ex vivofluorescence imaging of the tumour and normal tissues harvested from the euthanized MDA-MB-231 tumour-bearing nude mice at 24 h post injection. The numeric label for each organ is as follows: 1, heart; 2, liver; 3, spleen; 4, lung; 5, kidney; 6, tumour. (c) Region-of-interest analysis of fluorescent signals from the tumours and normal tissues. Error bars indicated s.d. (n=3). *P<0.05 (two-tailed Student’st-test). (d) The MDA-MB-231 tumour growth curves after intravenous injection of different formulations of Dox at a dose of 2 mg kg−1. Error bars indicate s.d. (n=5). *P<0.05, **P<0.01 (two-tailed Student’st-test). (e) Representative images of the MDA-MB-231 xenograft tumours of the mice after treatment with the studied Dox formulations at Day 14. Arrows indicate the sites of tumours. (f) The body weight variation of MDA-MB-231 tumour-bearing mice during treatment. Error bars indicate s.d. (n=5). (g) Histological observation of the tumour tissues after treatment. The tumour sections were stained with hematoxylin and eosin. Scale bar is 100 μm. (h) Detection of apoptosis in the tumour tissues after treatment. The tumour sections were stained with fluorescein-dUTP (green) for apoptosis and Hoechst for nuclei (blue). Scale bar is 200 μm. Figure 5: Tumour targetability and antitumour activity. ( a ) In vivo fluorescence imaging of the MDA-MB-231 tumour-bearing nude mice at 1, 6 and 24 h after intravenous injection of Dox/Cy5.5-Complex (I), Dox/Cy5.5-NG (II) and Dox/Cy5.5-NG with pre-injection of free HA (III) at Cy5.5 dose of 30 nmol kg −1 . Arrows indicate the sites of tumours. ( b ) Ex vivo fluorescence imaging of the tumour and normal tissues harvested from the euthanized MDA-MB-231 tumour-bearing nude mice at 24 h post injection. The numeric label for each organ is as follows: 1, heart; 2, liver; 3, spleen; 4, lung; 5, kidney; 6, tumour. ( c ) Region-of-interest analysis of fluorescent signals from the tumours and normal tissues. Error bars indicated s.d. ( n =3). * P <0.05 (two-tailed Student’s t -test). ( d ) The MDA-MB-231 tumour growth curves after intravenous injection of different formulations of Dox at a dose of 2 mg kg −1 . Error bars indicate s.d. ( n =5). * P <0.05, ** P <0.01 (two-tailed Student’s t -test). ( e ) Representative images of the MDA-MB-231 xenograft tumours of the mice after treatment with the studied Dox formulations at Day 14. Arrows indicate the sites of tumours. ( f ) The body weight variation of MDA-MB-231 tumour-bearing mice during treatment. Error bars indicate s.d. ( n =5). ( g ) Histological observation of the tumour tissues after treatment. The tumour sections were stained with hematoxylin and eosin. Scale bar is 100 μm. ( h ) Detection of apoptosis in the tumour tissues after treatment. The tumour sections were stained with fluorescein-dUTP (green) for apoptosis and Hoechst for nuclei (blue). Scale bar is 200 μm. Full size image We have also evaluated the pharmacokinetics and biodistribution of the Dox solution, Dox/Complex and Dox/NG after intravenous injection into the MB-MDA-231 tumour-bearing mice by quantitatively detecting the Dox amounts in the plasma and different tissues, including heart, liver, spleen, lung, kidney and tumour. Dox/NG showed an enhanced blood persistence compared with the Dox solution and Dox/Complex ( Supplementary Fig. 13 ). The area under the plasma concentration versus the time curves, elimination half-life ( t 1/2 ) and mean residence time of Dox/NG were remarkably higher than those of the Dox solution and Dox/Complex, which suggested that Dox/NG was able to maintain a high Dox concentration in the systemic circulation within a prolonged period. In addition, Dox/NG rendered higher Dox accumulation in the tumour tissues compared with the Dox solution and Dox/Complex ( Supplementary Fig. 14 ). The Dox amount in the tumour tissues delivered by Dox/NG was 4.19- and 3.94-fold that of those delivered by the Dox solution and Dox/Complex at 24 h post injection. It was validated that the ATP-responsive nanogels had high tumour targetability due to a combination of passive and active targeting mechanisms. Next, the antitumour efficacy of Dox/NG was estimated in MDA-MB-231 tumour xenograft models. As shown in Fig. 5d , different Dox formulations had significant effects on inhibiting tumour growth compared with saline as a negative control after successive intravenous administration into the tumour-bearing mice. Both Dox/cNG and Dox/NG presented remarkably higher inhibition efficacy towards tumour growth than the Dox solution, which primarily resulted from the tumour targeting capability of these nanogels. More importantly, a noticeable difference in tumour-size inhibition between Dox/NG and Dox/cNG was observed ( Fig. 5d,e ), suggesting that the efficient intracellular delivery and ATP-triggered Dox release are of great importance to enhanced antitumour activity. The body weights of the mice had no significant change during the treatment of Dox/NG ( Fig. 5f ). The histologic images using hematoxylin and eosin staining showed that after applying Dox/NG, a massive cancer cell remission occurred in the tumour tissue ( Fig. 5g ) while producing no obvious pathological abnormalities in the heart, such as cardiomyopathy, the main toxic effect in Dox cancer treatment [50] ( Supplementary Fig. 15 ). Moreover, the images obtained using the in situ TUNEL assay showed the highest level of cell apoptosis in the tumour harvested from the mice treated with Dox/NG ( Fig. 5h ), indicating that the dominant inhibition activity of tumour growth was attributable in part to the increased apoptosis effect induced by Dox/NG. Collectively, these results verified that ATP-responsive Dox/NG efficiently accumulated at the tumour site, demonstrated effective intracellular transport and ATP-mediated drug release, and thereby achieved optimal antitumour efficacy in vivo . We have developed an ATP-responsive anticancer DDS consisting of a nanogel with DNA, protein and polysaccharide. Our nanocarriers show drug release properties correlated to ATP levels, which selectively release the encapsulated Dox at high ATP levels for enhanced biological specificity and therapeutic efficacy in cancer therapy. We anticipate that this strategy will provide new opportunities for utilizing ATP as a metabolic trigger, which can lead to the development of increasingly specific DDS. Here Dox was intercalated in the GC-rich pairs of the DNA motif; however, other drugs [51] , [52] , [53] could also be loaded into the DNA chain through their specific affinity and be released by ATP’s invasion. Alternatively, drugs can be encapsulated into nanocarriers ‘caged’ by ATP aptamer for reversibly controlling drug release on ATP’s trigger. Furthermore, the intracellular level of ATP can be tuned by directly delivering ATP molecule [54] , [55] or adjusting other metabolic elements’ concentration or activity, such as glucose level, hydrogen ion gradient and oxidative stress [56] , [57] , [58] . Materials All chemicals were purchased from Sigma-Aldrich unless otherwise specified, and were used as received. Hyaluronic acid (HA, 77 kDa) was purchased from Freda Biochem Co., Ltd. (Shandong, China). ATP aptamer, single-stranded cDNA of ATP aptamer, control aptamer, cDNA of control aptamer and Cy5.5-labelled cDNA of ATP aptamer were purchased from Integrated DNA Technologies, Inc. (Coralville, USA). Preparation and characterization of Dox-loaded nanogels Hundred microlitres of m -protamine (0.7 mg ml −1 ) was mixed with 100 μl of Dox/Duplex (0.85 mg ml −1 ) and incubated for 10 min. The complex (Dox/Complex) was added into 200 μl of m -HA (0.35 mg ml −1 ) solution with stirring, followed by adding glycerol dimethacrylate (GDA) (0.07 mg). Radical polymerization was photoinitiated by Irgacure 2959 (0.1%, w:v) under the exposure to the ultraviolet radiation at the intensity of c.a. 20 mV cm −2 for 60 s using a BlueWave 75 UV Curing Spot Lamp (DYMAX). Finally, the resulting Dox-loaded nanogels (Dox/NG) were obtained by washing with nuclease-free water using centrifugal filter units (3 K MWCO) (Millipore) to remove the excessive crosslinker and initiator. Dox/Cy5.5-NG was obtained by the same method described above, except that Cy5.5-labelled duplex (Cy5.5-Duplex) hybridized by ATP aptamer and Cy5.5-labelled cDNA were added into the components of the nanogels to achieve a final Cy5.5 concentration of 5 μM in Dox/Cy5.5-NG. The particle size and zeta potential were measured by the Zetasizer (Nano ZS, Malvern). For TEM characterization, Dox/NG was dropped onto a TEM copper grid (300 mesh) (Ted Pella) and then stained with 1% (w:v) phosphotungstic acid for 1 min. After air dry, the sample was observed by TEM (JEM-2000FX, Hitachi) operating at 80 kV. In vitro ATP-triggered Dox release Dox/NG (0.5 ml) with 14 μg of Dox was added into a dialysis tube (10 K MWCO) (Slide-A-Lyzer, Thermo Scientific) against 14 ml of the HEPES buffer solution (5 mM HEPES, 10 mM MgCl 2 , 137 mM NaCl) containing different concentrations of ATP, and gently shaken at 37 °C in a shaker (New Brunswick Scientific) at 100 r.p.m. At predetermined time intervals, the total buffer solution was withdrawn, followed by replacing with 14 ml of fresh buffer solution with the same ATP concentration. The fluorescence intensity of Dox released was measured at 596 nm with an excitation wavelength of 480 nm by a microplate reader (Infinite M200 PRO, Tecan). Cell culture MDA-MB-231 and MCF-7 cells were obtained from Tissue Culture Facility of UNC Lineberger Comprehensive Cancer Center and cultured in DMEM with 10% (v:v) fetal bovine serum (FBS), 100 U ml −1 penicillin and 100 μg ml −1 streptomycin in an incubator (Thermo Scientific) at 37 °C under an atmosphere of 5% CO 2 and 90% relative humidity. The cells were sub-cultivated approximately every 3 days at 80% confluence using 0.25% (w:v) trypsin at a split ratio of 1:5. ATP-dependent Dox release in the cells MDA-MB-231 cells (1 × 10 5 cells per well) were seeded in six-well plates. After culture for 48 h, the cells were incubated with Dox-loaded nanogels (2 μM Dox concentration) for 2 h at 37 °C. Then, the excessive nanogels were removed and the cells were incubated with fresh FBS-free culture medium at 37 °C for additional 2 h or 4 h. After washing the cells by 4 °C PBS twice, the fluorescence intensity of Dox in the cells were measured using flow cytometry (BD FACSCalibur). Low temperature (4 °C) and IAA were used to inhibit ATP production in the cells. The content of ATP in the cells was assayed by the ATPlite Assay Kit (Perkin Elmer). After cell incubation with Dox/NG (2 μM Dox concentration) for 2 h at 37 °C, the excessive nanogels were removed and the cells were incubated at 4 °C or with IAA (100 μM) at 37 °C for additional 2 h or 4 h. After washing the cells by 4 °C PBS twice, the fluorescence intensity of Dox in the cells was measured using flow cytometry (BD FACSCalibur). Intracellular trafficking MDA-MB-231 cells (1 × 10 5 cells per well) were seeded in a confocal microscopy dish (MatTek). After culture for 24 h, the cells were incubated with Dox/NG (2 μM Dox concentration) at 37 °C for 2 h, and then washed by 4 °C PBS twice, followed by incubation with fresh FBS-free culture medium for additional 0 h or 4 h. Subsequently, the cells were stained by LyosTracker Green (50 nM) (Life Technologies) at 37 °C for 30 min and Hoechst 33342 (1 μg ml −1 ) (Life Technologies) at 37 °C for 10 min. Finally, the cells were washed by 4 °C PBS twice and immediately observed using CLSM (LSM 710, Zeiss). In vitro cytotoxicity MDA-MB-231 or MCF-7 cells (1 × 10 4 cells per well) were seeded in 96-well plates. After culture for 24 h, the cells were exposed to the Dox solution and Dox-loaded nanogels with different concentrations of Dox for 24 h, followed by adding 20 μl of the MTT solution (5 mg ml −1 ). After 4 h of incubation, the medium was removed, and the cells were mixed with 150 μl of dimethyl sulphoxide. The absorbance was measured at a test wavelength of 570 nm and a reference wavelength of 630 nm by a microplate reader (Infinite M200 PRO, Tecan). Apoptosis assay Apoptosis of MDA-MB-231 cells was detected using the APO-BrdU TUNEL Assay Kit (Life Technologies) and Annexin V-FITC Apoptosis Detection Kit (BD Biosciences). The cells (1 × 10 5 cells per well) were seeded in six-well plates. After culture for 48 h, the cells were incubated with Dox-loaded nanogels for 12 h (Annexin V-FITC) or 20 h (TUNEL). The subsequent procedures were performed in accordance with the manufacturer’s protocol. For Annexin V-FITC apoptosis detection, the cells were analysed by flow cytometry (BD FACSCalibur), while for TUNEL assay the cells were observed by fluorescence microscope (IX71, Olympus). Animals and tumour xenograft models All animals were treated in accordance with the Guide for Care and Use of Laboratory Animals, approved by the Institutional Animal Care and Use Committee (IACUC) of North Carolina State University. To set up the tumour xenograft model, the female nude mice (6 weeks, J:NU, The Jackson Laboratory) were subcutaneously inoculated in the back with 1 × 10 7 MDA-MB-231 cells. The tumour size was monitored by a vernier caliper and the tumour volume ( V ) was calculated as V = L × W 2 /2, where L and W were the length and width of the tumour, respectively. In vivo imaging study When the tumours reached to 200–400 mm 3 , the mice were intravenously injected by Dox/Cy5.5-Complex and Dox/Cy5.5-NG at Cy5.5 dose of 30 nmol kg −1 . For HA competitive study, the mice were pre-injected by a high dose of free HA (50 mg kg −1 ), and after 30 min were injected by Dox/Cy5.5-NG. Images were taken on IVIS Lumina imaging system (Caliper, USA) at 1, 6 and 24 h post injection. After the 24 h scanning, the mice were euthanized. The tumours as well as major organs were harvested, weighed and subjected for ex vivo imaging. Region-of-interests were circled around the organs, and the fluorescence intensities were analysed by Living Image Software. In vivo antitumour efficacy The tumour-bearing mice were weighed and randomly divided into different groups when the tumour volume reached to 50 mm 3 . From Day 0, the mice were intravenously injected with Dox solution (2 mg kg −1 ), Dox-loaded nanogels (2 mg kg −1 ) and saline as a negative control every other day for 12 days, and meanwhile the tumour size was measured. At Day 14, the mice were euthanized, and the tumour as well as the heart were collected, weighed, washed with saline thrice and fixed in the 10% neutral-buffered formalin. For the hematoxylin and eosin staining, the formalin-fixed tumours and hearts were embedded in paraffin blocks and visualized by optical microscope (DM5500B, Leica). For the TUNEL apoptosis staining, the fixed tumour sections were stained by the In Situ Cell Death Detection Kit (Roche Applied Science) according to the manufacturer’s protocol. Hoechst 33342 was used for nuclear counterstaining. The stained tumour slides were observed by fluorescence microscope (IX71, Olympus). How to cite this article: Mo, R. et al . ATP-triggered anticancer drug delivery. Nat. Commun. 5:3364 doi: 10.1038/ncomms4364 (2014).